Genomic deletions disrupt nitrogen metabolism pathways of a cyanobacterial diatom symbiont Diatoms with symbiotic N 2 -fixing cyanobacteria are often abundant in the oligotrophic open ocean gyres. The most abundant cyanobacterial symbionts form heterocysts (specialized cells for N 2 fixation) and provide nitrogen (N) to their hosts, but their morphology, cellular locations and abundances differ depending on the host. Here we show that the location of the symbiont and its dependency on the host are linked to the evolution of the symbiont genome. The genome of Richelia (found inside the siliceous frustule of Hemiaulus ) is reduced and lacks ammonium transporters, nitrate/nitrite reductases and glutamine:2-oxoglutarate aminotransferase. In contrast, the genome of the closely related Calothrix (found outside the frustule of Chaetoceros ) is more similar to those of free-living heterocyst-forming cyanobacteria. The genome of Richelia is an example of metabolic streamlining that has implications for the evolution of N 2 -fixing symbiosis and potentially for manipulating plant–cyanobacterial interactions. Cyanobacteria form partnerships with taxonomically diverse hosts that are usually multicellular, and these symbioses are ubiquitous in terrestrial and aquatic environments [1] . Cyanobacteria are autotrophic microorganisms and some can convert dinitrogen (N 2 ) gas to ammonium. Two groups of understudied planktonic symbioses are the partnerships between marine diatoms and the heterocyst-forming cyanobacteria, Richelia intracellularis and Calothrix rhizosoleniae ( Fig. 1a–c ). 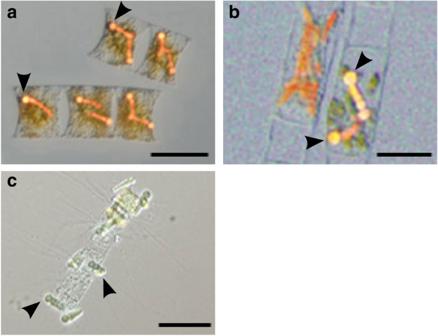Figure 1: Cyanobacteria in symbiosis with diatoms. Photomicrographs of cyanobacterial symbionts (denoted by arrows) representative of those sequenced in this study with host diatoms. Differential interference contrast bright field overlaid with blue light epifluorescence images of the diatomsH. membranaceus(a) andH. hauckii(b), with intracellular cyanobacterial symbionts. Bright-field microscopy image of epiphytic cyanobacterial symbiontC. rhizosoleniaeSC01 attached to the host diatomChaetocerossp. (c). Scale bars, 50 μm. Figure 1: Cyanobacteria in symbiosis with diatoms. Photomicrographs of cyanobacterial symbionts (denoted by arrows) representative of those sequenced in this study with host diatoms. Differential interference contrast bright field overlaid with blue light epifluorescence images of the diatoms H. membranaceus ( a ) and H. hauckii ( b ), with intracellular cyanobacterial symbionts. Bright-field microscopy image of epiphytic cyanobacterial symbiont C. rhizosoleniae SC01 attached to the host diatom Chaetoceros sp. ( c ). Scale bars, 50 μm. Full size image Richelia and Calothrix species convert N 2 and transfer the fixed N to their host [2] . Richelia and Calothrix associate with different hosts and also differ in cellular location (internal versus external), implying different life histories and mechanisms for nutrient exchanges with their partners. The Richelia symbionts of the diatom genera Rhizosolenia and Hemiaulus reside inside the diatom cell wall and are passed on to the next generation of the host [3] . The Rhizosolenia symbiont is outside the plasmalemma in the periplasmic space [3] ; the Hemiaulus symbiont’s location is unknown. In contrast, Calothrix attaches externally to Chaetoceros spp. and can be cultured without the host diatom in N-deplete media [4] . Reports of free-living Richelia may be a result of broken diatoms [5] , [6] , whereas Calothrix have been observed as individual trichomes in the plankton [7] , [8] . The mechanism of formation of a Calothrix – Chaetoceros association and whether the symbiont is transmitted to the next generation is unknown. We compared the genomes of two of the Richelia internal symbiont strains ( R. intracellularis HH01, RintHH, symbiont of Hemiaulus hauckii and R. intracellularis HM01, RintHM, symbiont of H. membranaceus ) with that of the external symbiont Calothrix rhizosoleniae SC01 (CalSC). We found that genome size and content, especially N metabolism genes, differed substantially, suggesting the cellular location (intracellular versus extracellular) has dictated varying evolutionary paths and resulted in different mechanisms involved in maintaining the symbiosis ( Table 1 ). Table 1 Nostocales genomes statistics. Full size table General features of the diatom symbiont genomes On the basis of the 16 rRNA and ntcA gene sequences, the diatom symbionts cluster within the cyanobacterial Order Nostocales ( Fig. 2 ), but their genome sizes vary greatly (RintHH, 3.2 Mb; CalSC, 6.0 Mb; Table 1 ). The percent coding information of the CalSC genome is only slightly lower than the free-living Nostocales members, whereas the RintHH genome percent coding is further reduced, similar to ‘ Nostoc azollae ’ 0708 ( Table 1 ). Similarly, the RintHH genome GC content and transporter count are lower than any other genome in the Order, whereas the CalSC genome is a more characteristic Nostocales genome in each respect ( Table 1 ). 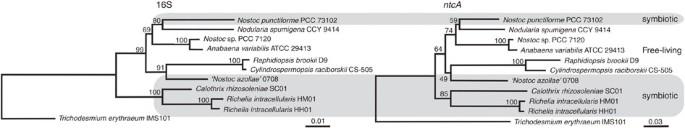Figure 2: Nostocales phylogeny. Neighbor-joining phylogenetic trees of 16S rRNA andntcAsequences from seven previously sequenced cyanobacteria and three additional diatom symbionts from this study. The organisms observed in symbiotic relationships are shaded in grey. Both trees are rooted withT. erythraeumIMS101. Locus tags (16S,ntcA): ‘N. azollae’ 0708 (Aazo_R0008, Aazo_1065),R. brookii(CRD_01297,CRD_00550),C. raciborskiiCS-505 (CRC_01246, CRC_00858),N. sp. PCC 7120 (allrr01, alr4392),N. spumigenaCCY9414 (N9414_r17988, N9414_19492),N. punctiformePCC 73102 (Npun_r020, Npun_F5511),A. variabilisATCC 29413 (Ava_R0006, Ava_3283),T. erythraeumIMS101 (Tery_R0014, Tery_2023),C. rhizosoleniaeSC01 (CSC01_11477, CSC01_6586),R. intracellularisHH01 (RintHH_r10, RintHH_12150),R. intracellularisHM01 (RintHM_3660, RintHM_9700). Figure 2: Nostocales phylogeny. Neighbor-joining phylogenetic trees of 16S rRNA and ntcA sequences from seven previously sequenced cyanobacteria and three additional diatom symbionts from this study. The organisms observed in symbiotic relationships are shaded in grey. Both trees are rooted with T. erythraeum IMS101. Locus tags (16S, ntcA ): ‘ N. azollae ’ 0708 (Aazo_R0008, Aazo_1065), R. brookii (CRD_01297,CRD_00550), C. raciborskii CS-505 (CRC_01246, CRC_00858), N . sp. PCC 7120 (allrr01, alr4392), N. spumigena CCY9414 (N9414_r17988, N9414_19492), N. punctiforme PCC 73102 (Npun_r020, Npun_F5511), A. variabilis ATCC 29413 (Ava_R0006, Ava_3283), T. erythraeum IMS101 (Tery_R0014, Tery_2023), C. rhizosoleniae SC01 (CSC01_11477, CSC01_6586), R. intracellularis HH01 (RintHH_r10, RintHH_12150), R. intracellularis HM01 (RintHM_3660, RintHM_9700). Full size image The genome of RintHM, the symbiont of H. membranaceus , a diatom that is closely related to H. hauckii , is only 2.2 Mb and is lacking a number of sequences expected of a full genome (including transfer RNAs for four amino acids and several nitrogenase genes). Therefore, we believe it is a partial genome, likely due to low-sequencing coverage (average depth of coverage 13 × ). However, 16S rRNA and ntcA sequences confirm the morphologically similar symbionts are also related genetically ( Fig. 2 ), as previously demonstrated by nifH and hetR sequences [9] , [10] . In addition, analysis of the contigs showed that there are no evident gene insertions/deletions or genome rearrangements between the two Hemiaulus sp. symbiont genomes. The 1,671 shared genes of the symbionts average 97.5% sequence identity (DNA) ( Supplementary Fig. S1 ) and show no significant difference in the GC content of the genes sequenced. Nitrogen metabolism of the diatom symbionts Given its small size, the RintHH genome is highlighted by many gene deletions, including numerous genes important in N metabolism, such as the transporters for ammonium and nitrate, and the genes encoding nitrate and nitrite reductases ( Fig. 3 ). The diatom symbiont genomes are each missing genes that encode urea transporters and urease, which are functional in all previously sequenced Nostocales genomes, except for the genome of ‘ N. azollae ’ 0708 (ref. 11 ). 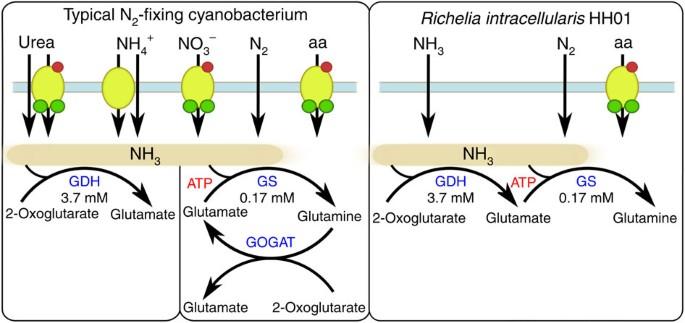Figure 3: Overview of the limited N pathways ofRichelia. Nitrogen metabolism pathways common in N2-fixing cyanobacteria compared withR. intracellularisHH01. Redrawn from33,34.Km-values for GDH and GS are for ammonia in each reaction from the N2-fixing cyanobacteriumSynechocystisPCC 6803 (refs18,35). Figure 3: Overview of the limited N pathways of Richelia . Nitrogen metabolism pathways common in N 2 -fixing cyanobacteria compared with R. intracellularis HH01. Redrawn from [33] , [34] . K m -values for GDH and GS are for ammonia in each reaction from the N 2 -fixing cyanobacterium Synechocystis PCC 6803 (refs 18 , 35 ). Full size image The most unusual gene deletion in RintHH is the gene for an important enzyme in C and N metabolism, glutamate synthase, also known as glutamine:2-oxoglutarate aminotransferase (GOGAT). This enzyme is part of glutamine synthetase (GS)-GOGAT (GS-GOGAT), a generally universal pathway for high-affinity N assimilation (found in all other sequenced cyanobacterial genomes [12] , including CalSC and ‘ N. azollae ’ 0708), which uses glutamine, synthesized by GS, and a C skeleton, 2-oxoglutarate, to produce two glutamate molecules. The glutamate produced by GOGAT is then recycled for further ammonium assimilation by GS. The gene encoding GS is present and functional in each symbiont genome; however, they are each lacking a gene that encodes a GS-inactivating factor that is found in all previously sequenced Nostocales genomes (asl2329 in Nostoc sp. PCC 7120). The multiple N metabolism genes missing from the RintHH genome are common to, and widely dispersed across, the genomes of all closed Nostocales genomes ( Supplementary Fig. S2 ). Given this, and the high-sequencing coverage of the RintHH draft genome (average depth of coverage >40 × ), it is unlikely that the missing genes are actually present in the RintHH genome. The RintHH genome does contain a tRNA for each of the 20 amino acids, as expected from a complete genome. Other sequences expected to be present are also in the assembly, such as the previously studied genes hetR and nifH [9] , [10] , and genes responsible for known characteristics of RintHH, such as nitrogen fixation, heterocyst formation, and phycoerythrin and chlorophyll pigments. Moreover, to decrease any possible bias during the process, two RintHH samples were separately sorted, amplified and sequenced. The majority of the N metabolism genes show no similarity to the RintHH genome. However, an intergenic sequence, which contains a small predicted hypothetical protein, has a top hit to the Raphidiopsis brookii GOGAT-encoding gene in the NCBI database of non-redundant (nr) protein sequences (BLASTx, E -value=3e −14 ; Fig. 4 ). The intergenic sequence covers less than 20% of the GOGAT gene and aligns in all three unidirectional frames. This intergenic region is found downstream of two genes that are part of a conserved region downstream of the GOGAT gene in Nostocales genomes. A single contig from the RintHM genome also shows similarity to the GOGAT gene in the same manner ( Fig. 4 ). 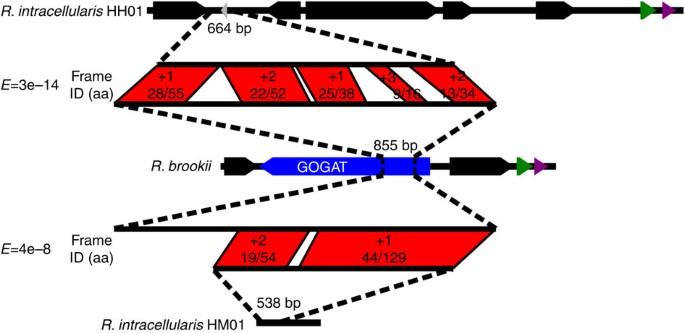Figure 4: GOGAT gene remnants inRichelia. The intergenic space between twoR. intracellularisHH01 ORFs, including an annotated 120 bp hypothetical protein (in grey, RintHH_15420) compared with the gene encoding GOGAT inRaphidiopsis brookiiD9 (in blue, CRD_00957) and the genomic context of each. The middle alignment represents the top BLAST hit of theR. intracellularisHH01 intergenic space (1561, bp) in the nr database (BLASTx,E-value=3e−14). The green and purple genes encode a mannose-6-phosphate isomerase and a probable iron binding protein, respectively. Figure 4: GOGAT gene remnants in Richelia . The intergenic space between two R. intracellularis HH01 ORFs, including an annotated 120 bp hypothetical protein (in grey, RintHH_15420) compared with the gene encoding GOGAT in Raphidiopsis brookii D9 (in blue, CRD_00957) and the genomic context of each. The middle alignment represents the top BLAST hit of the R. intracellularis HH01 intergenic space (1561, bp) in the nr database (BLASTx, E -value=3e−14). The green and purple genes encode a mannose-6-phosphate isomerase and a probable iron binding protein, respectively. Full size image Gene interruptions on the diatom symbiont nif operon The similarities with other heterocyst-forming cyanobacteria include the presence of insertion sequences in the middle of RintHH and CalSC N 2 -fixation genes [13] , [14] . The RintHH nifH gene is interrupted in this manner by a 9.1-kb sequence ( Fig. 5 ). The CalSC nifH and nifK genes are each interrupted in the same manner by longer sequences (each >20 kb). The nifH interruptions in RintHH and CalSC appear to occur at the same location within the nifH gene; however, the CalSC nifH element is at least twice as long as that in the RintHH genome. Recombination genes found on each nifH elements show high similarity to each other (71% ID, protein) and are presumably the mechanisms for excision of the element during heterocyst formation. 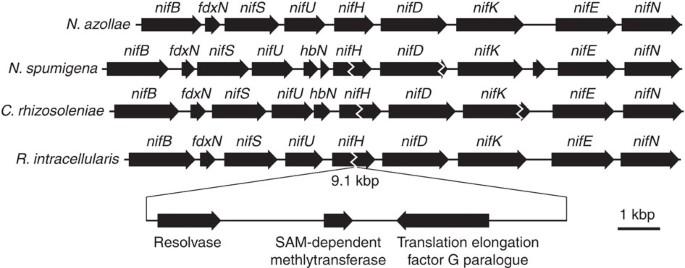Figure 5: Nitrogenase gene organization. Thenifoperon and surrounding genes ofR. intracellularisHH01 andC. rhizosoleniaeSC01 compared with other representative Nostocales cyanobacteria ‘Nostoc azollae’ 0708 andNodularia spumigenaCCY9414, and the genes along the insertion element interrupting theR. intracellularisHH01nifHgene. Figure 5: Nitrogenase gene organization. The nif operon and surrounding genes of R. intracellularis HH01 and C. rhizosoleniae SC01 compared with other representative Nostocales cyanobacteria ‘ Nostoc azollae ’ 0708 and Nodularia spumigena CCY9414, and the genes along the insertion element interrupting the R. intracellularis HH01 nifH gene. Full size image To date, the intracellular RintHH genome is the smallest N 2 -fixing, heterocyst-forming cyanobacteria genome sequenced. Within Nostocales, the R. brookii D9 genome is slightly smaller than that of RintHH, but it is unable to form heterocysts or fix N 2 (ref. 15 ). In contrast, the CalSC genome is similar in size and content to the genomes of free-living organisms in this Order and N. punctiforme , a facultative, or opportunistic, symbiont. The genome reduction in RintHH, marked by its size, percent coding and GC content, is similar to that of ‘ N. azollae ’ 0708, the obligate, or host-dependent, symbiont of the water fern Azolla filiculoides [11] . These features are commonly exhibited by genomes of obligate symbionts, indicating that RintHH is also dependent on its host. Obligate symbionts have more unnecessary genes than free-living or facultative symbiotic organisms due to metabolic redundancy encoded by the host genome and the lack of full exposure to the environment [16] . Examples of genes dispensable to obligate symbionts may be those absent or non-functional in both RintHH and ‘ N. azollae ’ 0708, but present in other heterocyst-forming cyanobacteria genomes ( Supplementary Table S1 ). Decreased evolutionary pressure to keep functional genes leads to a lower percent coding and eventually to genome size reduction as non-functioning genes are deleted. The smaller genome leads to accelerated sequence evolution, increasing AT bias [16] . The lack of CalSC genome reduction may be taken as evidence that this organism is an opportunistic partner. This is consistent with the external location of CalSC on the diatom setae (spine-like projections) and the ability to maintain it in culture independent of the host diatom in filtered seawater-based media [4] . In contrast, RintHH lives inside the host diatom cell wall, and possibly even within the cytoplasm, with little or no exposure to the external environment, and thus the genome reduction is consistent with that of an obligate symbiont. The numerous absent N metabolism genes appear to have been selectively deleted from multiple regions throughout the RintHH genome. The lack of ammonium transporters and enzymes required to take up and assimilate urea or nitrate limits the possible N sources for RintHH to amino acids, N 2 , and passive diffusion of ammonia in oceanic environments, where concentrations of amino acids and ammonium are extremely low. Therefore, deletions in N metabolism genes ensure N 2 fixation within the partner diatom persists, and is likely important for maintaining the symbiotic partnership. The lack of GOGAT, on the other hand, likely streamlines host–symbiont interactions and seems to be a more recent deletion than the other N metabolism genes, given the similarity between GOGAT genes and intergenic space in the RintHH genome. Without GOGAT, RintHH must use an alternate pathway for assimilation of N 2 -derived ammonium with glutamate dehydrogenase (GDH; Fig. 3 ), unless the host diatom provides glutamate for the symbiont. In contrast, GS-GOGAT is the main N assimilation pathway used by Anabaena azollae in obligate symbiosis with host Azolla caroliniana , and very little N is assimilated through GDH [17] . Given the high N 2 fixation rates by the cyanobacterial symbiont when associated with the host diatom [2] , it is feasible that intracellular ammonium concentrations are elevated and facilitate assimilation by the low-affinity GDH enzyme [18] . However, an adequate concentration of 2-oxoglutarate would also be needed to support ammonium assimilation. If these C skeletons are provided by the host, as in the Nostoc – Gunnera symbiosis [19] , the symbiont may perceive the increase of intracellular C:N as N starvation [20] , causing continued N 2 fixation by the cyanobacterium. Thus, the lack of GOGAT eliminates a common metabolic pathway and creates an N exchange pathway between host and symbiont that provides the host with a way to regulate the symbiont’s growth and activity. The lack of a GS-inactivating factor streamlines N metabolism further in RintHH. GS catalyses the conversion of glutamate to glutamine, and without an inactivating factor it will maintain low intracellular glutamate concentrations. The subsequent increasing glutamine pool may indicate this amino acid is the form of N passed to the host. The absence of this regulator shows parallels between the Richelia–Hemiaulus and Calothrix–Chaetoceros associations, and separates the diatom symbionts from other heterocyst-forming cyanobacteria. However, with regard to N metabolism, the similarities are minimal and the fundamental differences between the RintHH and CalSC genomes reflect the evolutionary selection of their metabolic interactions and cellular locations with the partner diatom. The extracellular CalSC symbiont is exposed to the open ocean environment at all times, and can therefore use a suite of dissolved inorganic nitrogen sources, albeit at low concentrations. Furthermore, the CalSC genome possesses a gene to encode GOGAT and, thus, the symbiont is capable of assimilating N through the high-affinity GS-GOGAT, in addition to GDH. However, a scenario for enhancing N 2 fixation by C transfer from the diatom to the external symbiont CalSC, as hypothesized for the Richelia – Hemiaulus association, would require a direct host–symbiont transport system. Otherwise, the extracellular C would likely be diluted immediately and available to other microorganisms. Thus, the extracellular location of CalSC on Chaetoceros spp. likely requires different mechanisms for N metabolism and exchange than intracellular RintHH. The differences in genome content and metabolic potential reflect the differences between obligate and facultative symbionts. Many heterocyst-forming cyanobacteria have DNA sequences interrupting N 2 fixation-related genes in vegetative cells, which are excised during genome rearrangements coincident with heterocyst development [21] , but the functional significance and evolutionary origin of these elements are unknown. These interrupting sequences have been seen previously in several genes [13] , [14] , [22] , but the CalSC genome is the first example of a nifK element. The location of elements within nifH and high similarity between the genes likely responsible for the excision of the interrupting sequence are the only apparent similarities between the two nifH elements in these closely related cyanobacteria. Although their similarities indicate the nifH elements in each organism have the same evolutionary origin, there seems to be little evolutionary pressure on the contents and length of the element. The characteristics of the genomes of symbiotic heterocyst-forming cyanobacteria reflect the differences in cellular location and host dependency. The absence of basic N metabolism enzymes and transporters in the RintHH genome streamline it, while maintaining the association and providing a mechanism for host regulation of the symbiont. In contrast, the genome of CalSC has few deletions relative to free-living heterocyst-forming cyanobacteria. The differences between genomes suggest mechanisms that may be important in defining facultative or obligate symbioses, with implications for the biology and ecology of these widespread symbiotic associations in the sea. Furthermore, differences in the genomic composition of morphologically and taxonomically similar microorganisms provides an important example of how one partner’s metabolic capabilities can evolve with a symbiosis. Finally, the genomes reported in this study, in addition to other recent discoveries of extensive metabolic streamlining in N 2 -fixing cyanobacteria [23] , yield the possibility of yet undiscovered plants or algae containing N 2 -fixing organelles. H. hauckii and H. membranaceus symbiont DNA preparation Stable Hemiaulus–Richelia cultures, isolated from the western Gulf of Mexico, were grown in N-free YBC-II medium at 25 °C (ref. 24 ), filtered on to a 3-μm pore size, 25-mm diameter polyester filter (Sterlitech) and frozen for storage. TE buffer (1 × ) was added, and once the filter thawed the cells were resuspended by vortexing for 1 min. The majority of diatoms were broken at this stage, releasing the symbionts in the process. Samples were then analysed on the Influx flow cytometer and cell sorter (BD Biosciences), and cyanobacteria cells were distinguished from other cells by their phycoerythrin pigmentation ( Fig. 6 ). For the H. hauckii symbionts, the vegetative trichomes and heterocysts had separated during the sample preparation and the cells formed separate populations on the flow cytometer based on slightly different chlorophyll and phycoerythrin signatures ( Fig. 6 ). Sorting gates, defined by relative pigment values, allowed for the isolation of vegetative cells from the rest of the sample. Two replicate sorts of 5,000 symbiont vegetative trichomes (3–5 cells per trichome) were sorted. Genomic DNA in each sample was amplified by multiple displacement amplification using the Repli-g Midi kit (Qiagen). The manufacturer’s protocol for 0.5 μl of cell material was followed with one exception: after buffer D2 was added, the samples were incubated for 5 min at 65 °C and then put on ice for 1 min, instead of 10 min on ice without a 65 °C incubation. 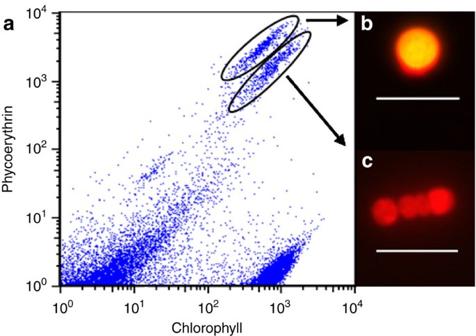Figure 6: Flow cytometric analysis ofR. intracellularis–H. hauckiiculture samples. A cytogram displaying events gated based upon chlorophyll (692/40 nm) and phycoerythrin (572/27 nm) detection channels with the cyanobacteria symbiont populations easily separated (a). Insets are microscopy images under blue excitation of a vegetative trichome (b) and a heterocyst cell (c) representative of circled populations. Scale bars, 10 μm. The vegetative trichome population was sorted for genome sequencing samples. Figure 6: Flow cytometric analysis of R. intracellularis–H. hauckii culture samples. A cytogram displaying events gated based upon chlorophyll (692/40 nm) and phycoerythrin (572/27 nm) detection channels with the cyanobacteria symbiont populations easily separated ( a ). Insets are microscopy images under blue excitation of a vegetative trichome ( b ) and a heterocyst cell ( c ) representative of circled populations. Scale bars, 10 μm. The vegetative trichome population was sorted for genome sequencing samples. Full size image To ensure uncontaminated samples, each amplified DNA sample was PCR-amplified using universal 16S rRNA primers 27F (5′-AGAGTTTGATCMTGGCTCAG-3′) and 1492R (5′-GGTTACCTTGTTACGACTT-3′) [25] . The PCR was carried out in 50 μl reactions consisting of 1 × PCR buffer, 2 mM MgCl 2 , 200 μM dNTPs, 0.2 μM of each primer and 1.5 U of Platinum Taq DNA polymerase (Invitrogen). A touchdown PCR was performed as follows: an initial denaturing step at 94 °C for 5 min, followed by 30 cycles of three 1-min steps (denaturation at 94 °C, annealing at 53–41 °C and elongation at 72 °C) and a final elongation step at 72 °C for 10 min. The first cycle annealing took place at 53 °C and was lowered by 0.4 °C for each cycle to reach 41 °C for the final cycle. Resulting products were run on a 1.2% agarose gel, the distinct bands of ~1,500 bp were excised and then recovered using the Zymoclean DNA Recovery Kit (Zymo Research). The recovered DNA was then ligated and plated for blue/white screening using the pGem-T and pGem-T Easy Vectors Systems (Promega). Twenty-four colonies per sample were picked and grown overnight at 37 °C in 2 × LB media with carbenicillin (200 μg ml −1 ). The Montáge Plasmid Miniprep HTS Kit (Millipore) was used following the manufacturer’s instructions for the full lysate protocol for plasmid DNA miniprep. Samples were sequenced at UC-Berkeley DNA Sequencing Facility and each sequence was subject to BLAST analysis against the nt database (BLASTn). All sequences were identical and had top hits to 16S rRNA sequences of heterocyst-forming cyanobacteria, confirming no contaminant genomes were present in the samples. DNA concentration and quality were checked (Agilent 2100 Bioanalyzer, Agilent Technologies) before submission for 454 Titanium sequencing (Roche) at the UCSC Genome Technology Center. The symbionts of H. membranaceus were processed in the same manner, but heterocysts and vegetative cells did not separate during sample preparation, and both cell types were present in the sorted samples. Moreover, we were confident from flow cytometry that the cell preparation was pure enough to determine the comparative features we were looking for, and that we would be able to distinguish between the closely related symbiont and the few bacteria that could be carried through by flow cytometry. Therefore, no contamination or DNA quality checks were performed in preparation of the RintHM samples. H. hauckii and H. membranaceus symbiont genome assembly A total of 433,028 reads were sequenced from RintHM samples. The reads assembled to nearly 8 Mb and the assembly contained four 16S rRNA sequences with low similarity to each other (<83% ID), indicating multiple DNA sources in the data. RintHM contigs were defined as those which had a better BLAST hit to RintHH than to any other organism in the nt database. The resulting 2,212,909 bp (941 contigs, coverage depth 13 × ) were made up of 77,324 reads averaging 380 bp each. An additional 31 contigs, totalling 97,821 bp, had a top hit in the nt database to a cyanobacterium other than RintHH, but none of those contigs contained any of the N metabolism genes of interest. The two RintHH samples yielded a total 409,035 reads, averaging 344 bp each. The read data were pooled and assembled into 3,243,759 bp in 90 contigs (coverage depth 43 × ) and appeared to be non-contaminated. There are seven contigs longer than 100 kbp, an additional 32 contigs longer than 25 kbp ( Supplementary Fig. S3 ) and 91% of bases with 15 × coverage or greater. CalSC DNA preparation CalSC genomic DNA was extracted from pelleted cells using a sucrose lysis protocol, including the optional back extraction [26] . The exceptions to this protocol were our use of 10% SDS in the lysate for Fraction B instead of 20% SDS and the 1-h incubation of Fraction B after adding the lysate was at 37 °C rather than 55 °C. The genomic DNAs from Fraction B were pooled and divided into three equal volume samples. The three genomic extracts were checked for purity and quantity (Agilent 2100 Bioanalyzer, Agilent Technologies), and the DNA concentrations ranged between 38.37 and 66.38 ng μl −1 . Samples were then submitted to JCVI for 454 sequencing. CalSC genome assembly Once the read data from JCVI (2,477,040 reads, 968 MB) were assembled, the number of contigs (69,919) and size of the assembly (81.4 Mb) immediately suggested that more than one organism was in the sequencing samples. The longest contig of 1.2 MB in length contained a full-length rRNA operon predicted by RDP (Ribosomal Database Project) to be a Planctomycete, confirming the presence of organisms other than CalSC. A plot of the number of reads on each contig against the length of the contig showed strong linear relationships ( Supplementary Fig. S4 ), representing defined clusters of coverage depth, based on the relative abundance of the each organism’s genome in the sample. Spot-checking the phylogeny of BLASTn results for long open reading frames (ORFs) on long contigs revealed that the contigs lying along the line marked in red (representing a coverage depth of 30 × ) were those that came from CalSC ( Supplementary Fig. S4 ). Each predicted ORF >450 bp on contigs with depth of coverage 15–45 × was subject to BLAST analysis against the nt database. A contig was considered to be part of the CalSC genome if at least one of these ORFs on the contig had a top hit to a cyanobacterial sequence, and 471 contigs met this criterion (5,967,587 bp). One additional contig (5,416 bp) containing the rRNA operon was added. It had been overlooked initially due to its lack of ORFs and its relatively higher coverage depth (71 × , indicating it is present in two copies in the genome). The end result was a 5,973,003 bp genome composed of 472 contigs (30 × coverage depth). Genomic analysis After assembly and contamination screening, the genomes were submitted to RAST (Rapid Annotation using Subsystem Technology) [27] for annotation. The nitrogen metabolism genes not found in the RintHH genome were pulled from each Nostocales genome, and each gene was subject to BLAST analysis against a database of all 409,035 reads (tBLASTn, e <10). Two thousand seven hundred and twenty reads had hits at least 25% identical (AA) across at least 50% the length of the read or gene, whichever was shorter. A BLAST analysis of each of these reads against the nr database was performed (BLASTx, e <10). Twenty-one reads had a top hit to a GOGAT-encoding gene, and each of these reads is assembled into the intergenic region discussed below as likely GOGAT remnants in the RintHH genome. No other reads had a top hit in the nr database of a nitrogen metabolism-related gene. Predicted ORFs in each genome with a BLAST hit in the Transporter Classification database [28] (BLASTp, E -value <1E−19) were counted as transporter genes. For the 16S rRNA and the ntcA phylogenetic trees, nucleotide sequences were acquired from DOE Joint Genome Institute for each of the seven previously sequenced Nostocales genomes and Trichodesmium erythraeum IMS101, and were aligned with the sequences from the three diatom symbiont genomes using Clustal W [29] (1,421 bp, 16S rRNA; 646 bp, ntcA ). Phylogenetic analyses were rendered in Mega5 (ref. 30 ) using the Neighbor-Joining method [31] . The Tamura–Nei test was run to detect the best models. Statistical support for nodes was based on 1,000 bootstrap replicates [32] . Accession codes: The genomes described in this study have been deposited at the European Nucleotide Archive (ENA) under accession numbers CAIY01000001 to CAIY01000090 (RintHH) , CAIS01000001 to CAIS01000941 (RintHM) and SRX023670 (CalSC) . How to cite this article: Hilton, J. A. et al . Genomic deletions disrupt nitrogen metabolism pathways of a cyanobacterial diatom symbiont. Nat. Commun. 4:1767 doi: 10.1038/ncomms2748 (2013).